Structural analysis and mapping of individual protein complexes by infrared nanospectroscopy Mid-infrared spectroscopy is a widely used tool for material identification and secondary structure analysis in chemistry, biology and biochemistry. However, the diffraction limit prevents nanoscale protein studies. Here we introduce mapping of protein structure with 30 nm lateral resolution and sensitivity to individual protein complexes by Fourier transform infrared nanospectroscopy (nano-FTIR). We present local broadband spectra of one virus, ferritin complexes, purple membranes and insulin aggregates, which can be interpreted in terms of their α-helical and/or β-sheet structure. Applying nano-FTIR for studying insulin fibrils—a model system widely used in neurodegenerative disease research—we find clear evidence that 3-nm-thin amyloid-like fibrils contain a large amount of α-helical structure. This reveals the surprisingly high level of protein organization in the fibril’s periphery, which might explain why fibrils associate. We envision a wide application potential of nano-FTIR, including cellular receptor in vitro mapping and analysis of proteins within quaternary structures. Fourier transform infrared spectroscopy (FTIR) allows for the analysis of chemical bonds, protein morphology or secondary structure [1] , [2] , [3] , [4] . Applications include the tracing of protein modifications that may originate from interactions with other biomaterials (for example, cellular receptors and enzymatic cofactor) [5] or inorganic matter (for example, heavy metal ions and nanoparticles) [6] . Such interactions are of high relevance in various physiological cellular processes (for example, cellular attachment and genomic regulation), pathological processes of a large variety of diseases (for example, viral infection and neurodegenerative diseases) [7] , [8] , as well as in biomedical diagnostics and equipment (for example, support for human cell culture) [9] . The analysis of amide vibrations provides valuable insights into the secondary structures of proteins, revealing information regarding conformation and folding [3] , [10] , [11] , [12] , [13] . However, because of the diffraction-limited resolution of FTIR, infrared spectroscopy applications on the nanometre scale or even single-molecule level have so far proved elusive. The diffraction-limited resolution of FTIR is circumvented by Fourier transform infrared nanospectroscopy (nano-FTIR) [14] , [15] , [16] , [17] , [18] , [19] . This technique is based on scattering-type scanning near-field optical microscopy (s-SNOM) [20] where infrared images with nanoscale spatial resolution are obtained by recording the infrared light scattered at a scanning probe tip. The probe is typically a metalized atomic force microscope (AFM) tip. Acting as an antenna, it concentrates the incident field at the tip apex [15] , [20] for local probing of molecular vibrations, similar to tip-enhanced Raman spectroscopy [21] , [22] , [23] , [24] . When the AFM tip is illuminated by the broadband infrared radiation, Fourier transform spectroscopy of the scattered light yields infrared spectra with a spatial resolution down to 20 nm (refs 16 , 17 , 18 , 19 ). However, broadband nano-FTIR spectra of protein complexes have neither been observed so far nor shown to be suitable for the analysis of their structure. Biological objects such as protein fibrils and membranes have been already studied by s-SNOM imaging at selected wavelengths [25] , [26] , [27] , [28] , [29] but it has not been demonstrated that the most important secondary structures—α-helical and β-sheet structures—can be identified on the level of individual protein complexes. To demonstrate that nano-FTIR can probe protein secondary structure on the nanometre scale and with sensitivity to individual protein complexes, we have chosen to study the amide bands of individual tobacco mosaic viruses (TMVs) and ferritin complexes [30] for their well-defined, robust and dominantly α-helical protein structure [31] , insulin aggregates for exhibiting β-sheet structure [32] and purple membranes (PMs) because of the well-defined orientation of the transmembrane α-helices [33] . Broadband infrared spectra of a ferritin complex indicate that nano-FTIR is sensitive to about 4,000 amino acids, corresponding to about 5,000 C=O and N-H bonds, respectively. Most importantly, we find that the amide I band in the nano-FTIR spectra can be analysed and interpreted in the framework of standard infrared spectroscopy. Our studies establish a solid foundation for infrared nanobiospectroscopy, which is a prerequisite for nano-FTIR applications in biochemical and biomedical research. We demonstrate the potential for real-life applications of nano-FTIR in these fields by exploring the still not fully clarified protein conformation in individual insulin fibrils. s-SNOM and nano-FTIR set-up The s-SNOM and nano-FTIR set-up (Neaspec GmbH, Germany) used in this work is based on an AFM where the tip is oscillating vertically at the mechanical resonance frequency Ω of the cantilever. Infrared near-field imaging and spectroscopy are performed by interferometric detection of the light scattered from a gold-coated AFM tip, which is illuminated by the radiation from a tunable quantum cascade laser (QCL) or a broadband mid-infrared laser beam, respectively ( Fig. 1a,b ). 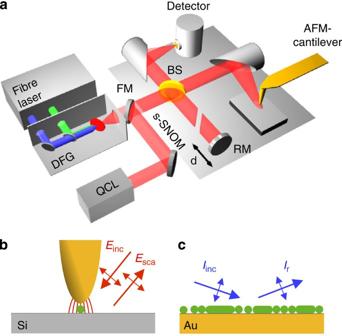Figure 1: Infrared spectroscopy of protein nanostructures. (a) s-SNOM and nano-FTIR set-up employing a tunable single line laser (quantum cascade laser, QCL) or a mid-infrared continuum source (fibre laser plus difference frequency generator) for tip illumination, respectively. The illumination can be chosen with a flip mirror (FM). The light backscattered from the tip is analysed with a Michelson interferometer that is operated in either pseudoheterodyne mode (for s-SNOM imaging) or as a Fourier transform spectrometer (for nano-FTIR spectroscopy). It comprises a beam splitter (BS, uncoated ZnSe), a reference mirror (RM) and a detector. (b) Schematics of s-SNOM and nano-FTIR spectroscopy. (c) Schematics of far-field GI-FTIR spectroscopy of protein nanostructure ensembles. Figure 1: Infrared spectroscopy of protein nanostructures. ( a ) s-SNOM and nano-FTIR set-up employing a tunable single line laser (quantum cascade laser, QCL) or a mid-infrared continuum source (fibre laser plus difference frequency generator) for tip illumination, respectively. The illumination can be chosen with a flip mirror (FM). The light backscattered from the tip is analysed with a Michelson interferometer that is operated in either pseudoheterodyne mode (for s-SNOM imaging) or as a Fourier transform spectrometer (for nano-FTIR spectroscopy). It comprises a beam splitter (BS, uncoated ZnSe), a reference mirror (RM) and a detector. ( b ) Schematics of s-SNOM and nano-FTIR spectroscopy. ( c ) Schematics of far-field GI-FTIR spectroscopy of protein nanostructure ensembles. Full size image For s-SNOM imaging, the tip is illuminated with radiation from the wavelength-tunable QCL at individual wavelengths. The tip-scattered light is detected by operating the interferometer in pseudoheterodyne mode [34] . Demodulating the detector signal at a higher harmonic n Ω of the tip oscillation frequency yields infrared amplitude and phase images, s n and ϕ n (see Methods section). In nano-FTIR spectroscopy, broadband infrared amplitude and phase spectra are obtained by employing the interferometer for Fourier transform spectroscopy of the scattered light [14] , [15] , [16] , [17] , [18] , [19] . In this case, the tip is illuminated with a broadband laser of a total power of about 100 μW (refs 17 , 35 ). As the tip and the sample are located in one of the interferometer arms (in contrast to standard FTIR), we can measure both local amplitude and phase spectra, s n ( ω ) and ϕ n ( ω ). These spectra are normalized to the references, s ref ,n ( ω ) and ϕ ref ,n ( ω ), obtained on a clean area on the sample support (marked R in the topography images presented in the work). We thus obtain normalized amplitude and phase spectra form which we can calculate the nano-FTIR absorption spectrum a n ( ω )= s n / s ref ,n sin ( ϕ n − ϕ ref ,n ). As demonstrated in refs 17 , 19 , the nano-FTIR spectrum a n ( ω ) reveals the local infrared absorption in the sample. Setting the foundations for protein analysis with nano-FTIR We first verify the ability of nano-FTIR to measure nanoscale broadband infrared spectra of the amide I and II bands over the range from 1,400 to 1,800 cm −1 . To that end, we studied TMVs ( Fig. 2a ). These well-defined protein complexes have a diameter of 18 nm and a length of 300 nm, and consist of 2,140 identical proteins assembled helically around an RNA strand [31] . 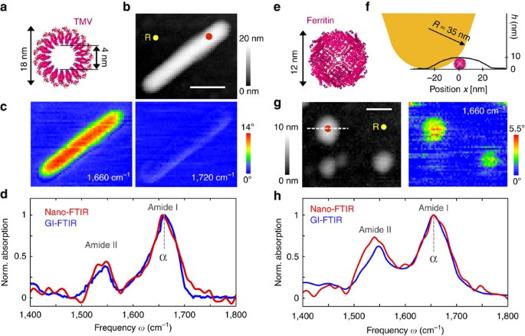Figure 2: Infrared nanospectroscopy of TMV and individual ferritin protein complexes. (a) Illustration of the protein structure of TMV. (b) Topography of TMV on a silicon substrate. Scale bar, 100 nm. (c) Infrared near-field phase imagesϕ3at two different frequencies, 1,660 cm−1(left) and 1,720 cm−1(right; 2.5 min total image acquisition time). (d) Nano-FTIR spectrum of TMV taken at the position marked by the red dot in the topography image (red, average of 40 interferograms; 22 min total acquisition time; 8 cm−1resolution; × 4 zero filling) and a GI-FTIR spectra of a large TMV ensemble on a gold substrate (blue). (e) Illustration of the protein structure of ferritin. (f) Illustration of the tip probing a ferritin particle. The graph shows the measured height profilehwhen the tip is scanned along the dashed line inFig. 2g. (g) Topography and infrared near-field imageϕ3of two ferritin molecules and a ferrihydrite core on a silicon substrate. Scale bar, 50 nm (1.5 min total image acquisition time). (h) Nano-FTIR (red) and GI-FTIR spectra of a large ferritin ensemble on a gold substrate (blue). The red dot in the topography image marks the position where the nano-FTIR spectra (average of 60 interferograms; 23 min total acquisition time; 8 cm−1resolution; × 4 zero filling) was recorded. The position marked by the yellow dot and R inbandgindicates where the reference spectrum was recorded. Figure 2c shows near-field infrared phase ϕ 3 images taken at 1,660 and 1,720 cm −1 , that is, on and off resonance with the amide I vibration. At 1,660 cm −1 , the phase image exhibits strong contrast owing to the amide I absorption [25] . As expected, the phase contrast vanishes when the illumination is tuned to 1,720 cm −1 where the protein does not absorb. From nano-FTIR amplitude s 3 ( ω ) and phase ϕ 3 ( ω ) spectra recorded on top of the virus (position marked by the red dot in the topography image) and normalized to those taken on a clean silicon area, we obtained the local infrared absorption spectrum a 3 (red spectrum in Fig. 2d ). For comparison, we recorded a FTIR spectrum of a large TMV ensemble (blue spectrum in Fig. 2d ) by employing p -polarized-grazing incidence (GI-FTIR, schematics see Fig. 1c ). We find a good agreement between the GI-FTIR and nano-FTIR spectra. Both reveal the amide I and amide II bands associated with combinations of C=O and C-N stretching with C-N-H-bending vibrations, respectively. We note that the agreement can vary among different amide bands, since the exact peak position and shape of an absorption band depend on the band strength and the employed FTIR technique [36] (see also Supplementary Fig. S1 ). Figure 2: Infrared nanospectroscopy of TMV and individual ferritin protein complexes. ( a ) Illustration of the protein structure of TMV. ( b ) Topography of TMV on a silicon substrate. Scale bar, 100 nm. ( c ) Infrared near-field phase images ϕ 3 at two different frequencies, 1,660 cm −1 (left) and 1,720 cm −1 (right; 2.5 min total image acquisition time). ( d ) Nano-FTIR spectrum of TMV taken at the position marked by the red dot in the topography image (red, average of 40 interferograms; 22 min total acquisition time; 8 cm −1 resolution; × 4 zero filling) and a GI-FTIR spectra of a large TMV ensemble on a gold substrate (blue). ( e ) Illustration of the protein structure of ferritin. ( f ) Illustration of the tip probing a ferritin particle. The graph shows the measured height profile h when the tip is scanned along the dashed line in Fig. 2g . ( g ) Topography and infrared near-field image ϕ 3 of two ferritin molecules and a ferrihydrite core on a silicon substrate. Scale bar, 50 nm (1.5 min total image acquisition time). ( h ) Nano-FTIR (red) and GI-FTIR spectra of a large ferritin ensemble on a gold substrate (blue). The red dot in the topography image marks the position where the nano-FTIR spectra (average of 60 interferograms; 23 min total acquisition time; 8 cm −1 resolution; × 4 zero filling) was recorded. The position marked by the yellow dot and R in b and g indicates where the reference spectrum was recorded. Full size image In Fig. 2e–h , we perform nano-FTIR studies of ferritin, a globular protein complex of 12 nm in diameter. Ferritin comprises 24 subunits that form a cage around a ferrihydrite nanoparticle ( Fig. 2e ). Each ferritin subunit is composed of six α-helixes and one β-sheet [30] . The topographical image in Fig. 2g shows two particles of about 10 and 8 nm, and one of about 6 nm height, which appear much broader because of the convolution with tip apex that has a radius of about 35 nm (see Fig. 2f and Supplementary Fig. S2 ). The infrared phase image ϕ 3 at 1,660 cm −1 reveals a strong absorption for the 10- and 8-nm particles, indicating that these are ferritin complexes. No infrared contrast is seen for the 6-nm particle, which we interpret as ferrihydrite core that does not absorb at 1,660 cm −1 . Figure 2h shows the nano-FTIR spectrum (red curve) of the ferritin marked by the red dot in Fig. 2g in comparison with a GI-FTIR spectrum of a large ferritin ensemble (blue curve). As demonstrated with the TMV ( vide supra ), the nano-FTIR spectrum reveals the amide I and II bands in excellent agreement with GI-FTIR. Thus, we conclude that nano-FTIR allows for measuring infrared spectra of individual protein complexes, which can be interpreted by comparison with standard GI-FTIR absorbance spectra. The analysis provided in Supplementary Fig. S2 and Supplementary Note 1 indicates that the marked object is one ferritin complex. To explore whether and how nano-FTIR absorption spectra depend on the protein orientation, we studied the PMs of Halobacterium salinarum ( Fig. 3 ), which is composed of a double layer of polar and neutral lipids, and the integral membrane protein bacteriorhodopsin. The secondary structure of bacteriorhodopsin comprises seven transmembrane α-helices and an extracellular β-sheet [33] . As the helices are predominantly oriented perpendicular to the membrane plane, the infrared amide I vibration is normal to the membrane surface, whereas the amide II vibration is parallel to the membrane surface [37] (see illustration in Fig. 3b ). The well-defined directions of the amide vibrations render PM an excellent protein structure for studying the sensitivity of nano-FTIR to protein orientation. In the topography image ( Fig. 3a ), the membranes appear as 6 nm high flat layers. As before with the TMV, the infrared phase contrast ( Fig. 3c ) at 1,660 cm −1 exhibits the typical amide I absorption, which vanishes at 1,720 cm −1 because the archaeobacterial PM is devoid of any ester lipids that usually give rise to carbonyl stretching vibrations in lipid membranes of eubacteria and eukarya. A nano-FTIR spectrum a 3 ( Fig. 3d , red curve) is obtained by placing the tip atop the PM (marked by red dot in Fig. 3a ), analogous to the TMV experiment. The GI-FTIR spectrum ( p -polarized incident field) of horizontally adsorbed PMs was recorded for comparison ( Fig. 3d , blue curve; for schematics see Fig. 1c ). Interestingly, the amide II band does not appear in both spectra. In the GI-FTIR experiment, the electric field is perpendicular to the PM surface and thus perpendicular to the direction of the amide II vibrations. For that reason, amide II vibrations are not excited [37] . The absence of the amide II band in the nano-FTIR spectrum is explained by the field distribution at the tip apex, which essentially is that of a vertically oriented point dipole located in the tip apex ( Fig. 3b ) [20] . The strongest field, located directly below the tip apex, is vertically oriented, and efficiently couples the protein vibrations normal to the PM surface (amide I) but not the protein vibrations parallel to the PM surface (amide II). This orientation-dependent effect is well known from surface-enhanced IR absorption spectroscopy [38] . Thus, we conclude that nano-FTIR primarily probes molecular vibrations that oscillate perpendicular to the sample surface. 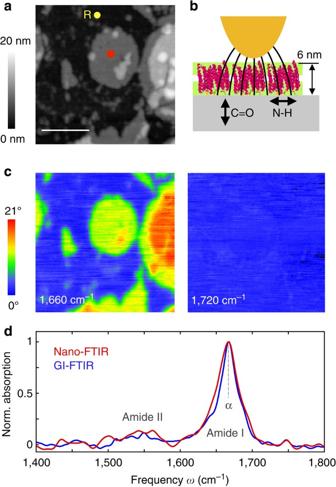Figure 3: Nano-FTIR sensitivity to protein orientation demonstrated with PM. (a) Topography of PMs on a silicon substrate. Scale bar, 400 nm. (b) Illustration of near-field probing of PM. (c) Infrared near-field phase imagesϕ3at two different frequencies, 1,660 cm−1(left) and 1,720 cm−1(right; 19 min total image acquisition time). (d) Nano-FTIR (red) and GI-FTIR spectra of an ensemble of horizontally absorbed PMs on a gold substrate (blue). The red dot in the topography image marks the position where the nano-FTIR spectra (average of 60 interferograms; 23 min total acquisition time; 8 cm−1resolution; × 4 zero filling) was recorded. The position marked by the yellow dot and R indicates where the reference spectrum was recorded. Figure 3: Nano-FTIR sensitivity to protein orientation demonstrated with PM. ( a ) Topography of PMs on a silicon substrate. Scale bar, 400 nm. ( b ) Illustration of near-field probing of PM. ( c ) Infrared near-field phase images ϕ 3 at two different frequencies, 1,660 cm −1 (left) and 1,720 cm −1 (right; 19 min total image acquisition time). ( d ) Nano-FTIR (red) and GI-FTIR spectra of an ensemble of horizontally absorbed PMs on a gold substrate (blue). The red dot in the topography image marks the position where the nano-FTIR spectra (average of 60 interferograms; 23 min total acquisition time; 8 cm −1 resolution; × 4 zero filling) was recorded. The position marked by the yellow dot and R indicates where the reference spectrum was recorded. Full size image In Fig. 4 , we evaluate the spatial resolution and reproducibility of nano-FTIR protein spectroscopy by recording 20 spectra, while the tip is scanning in steps of 10 nm across the PM. The spectral line scan ( Fig. 4b ) along the line of red and blue dots in the topography image ( Fig. 4a ) reveals the amide I peak on top of the membrane until the edge is reached (at position x ≈80 nm). Plotting the nano-FTIR absorption a 3 at 1,660 cm −1 as a function of the position x ( Fig. 4c ) shows that absorption vanishes within three scan steps. This demonstrates a spatial resolution of about 30 nm, which is an improvement by more than 100 compared with micro-FTIR mapping [39] . We further note that the eight local infrared spectra on the PM (P1–P8, between x =0 and 70 nm) exhibit a stable peak position and peak height, which illustrates the high reproducibility of nano-FTIR ( Fig. 4d ). On the other hand, these results show that the infrared absorption of PM does not exhibit significant spatial variations, confirming the homogeneity of the protein structure within the PM. 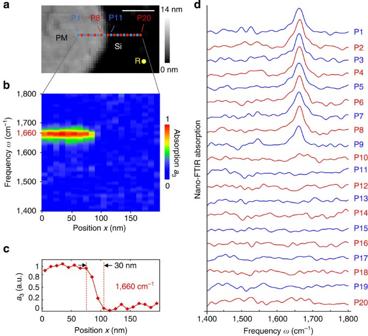Figure 4: Nano-FTIR mapping of PM. (a) Topography image of PM on a silicon substrate. Scale bar, 100 nm. (b) Infrared spectroscopic line scan recorded while the tip was scanned in 10 nm steps along the line of red and blue dots ina. At the position of each dot, a spectrum was taken (each spectrum is an average of 17 interferograms; 2.3 min acquisition time; 16 cm−1resolution; × 6 zero filling). (c) Absorption signala3at 1,660 cm1as a function of positionx. (d) Twenty nano-FTIR spectra recorded at the positions P1–P20 marked by red and blue dots ina. The spectra are the same as those presented inb. For better visibility, each spectrum is vertically offset. All spectra have been normalized to the reference spectrum recorded at the position marked by the yellow dot and R ina. Figure 4: Nano-FTIR mapping of PM. ( a ) Topography image of PM on a silicon substrate. Scale bar, 100 nm. ( b ) Infrared spectroscopic line scan recorded while the tip was scanned in 10 nm steps along the line of red and blue dots in a . At the position of each dot, a spectrum was taken (each spectrum is an average of 17 interferograms; 2.3 min acquisition time; 16 cm −1 resolution; × 6 zero filling). ( c ) Absorption signal a 3 at 1,660 cm 1 as a function of position x . ( d ) Twenty nano-FTIR spectra recorded at the positions P1–P20 marked by red and blue dots in a . The spectra are the same as those presented in b . For better visibility, each spectrum is vertically offset. All spectra have been normalized to the reference spectrum recorded at the position marked by the yellow dot and R in a . Full size image Nanoscale mapping of structural protein heterogeneity To establish nanoscale identification of α-helical and β-sheet structure in proteins, and to demonstrate heterogeneity in a sample at the nanometre scale that is only resolvable by nano-FTIR, we studied insulin aggregates deliberately contaminated with a low amount of TMV ( Fig. 5 ). While α-helices dominate in TMV, the insulin aggregates are composed of essentially two β-sheets [32] . The TMV can be thus considered a diluted α-helical structure within a β-sheet sample. Note that for sample preparation, we used a 2-year old insulin solution (see Methods section) because we found that such a solution yields insulin aggregates rather than well-defined fibrils. For such a sample, we expect that the orientation of the infrared-active β-sheet dipole of the amide I band is random, thus yielding a signal in nano-FTIR. Note that only vertically oriented dipoles yield a signal in nano-FTIR (see Fig. 3 ). 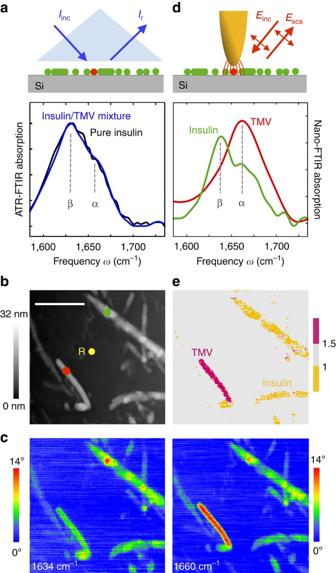Figure 5: Nanoscale mapping of α-helical and β-sheet secondary structure. (a) ATR-FTIR spectrum of a pure insulin aggregate sample (black) and a mixture of insulin aggregates and TMV (blue) on a silicon support. (b) Topography of a mixture of TMV and insulin aggregates on silicon. Scale bar, 500 nm. (c) Infrared near-field phase imagesϕ3at two different frequencies, 1,634 cm−1(left) and 1,660 cm−1(right; 19 min total image acquisition time). (d) Nano-FTIR spectra of TMV (red, average of 70 interferograms; 19 min total acquisition time; 16 cm−1resolution; × 4 zero filling) and insulin aggregate (green, average of 40 interferograms; 22 min total acquisition time; 8 cm−1resolution × 4 zero filling). Red and green dots in the topography image mark the positions where the nano-FTIR spectra were taken. The position marked by the yellow dot and R indicates where the reference spectrum was recorded. (e) Map of TMV (purple) and insulin (yellow) aggregates. Figure 5: Nanoscale mapping of α-helical and β-sheet secondary structure. ( a ) ATR-FTIR spectrum of a pure insulin aggregate sample (black) and a mixture of insulin aggregates and TMV (blue) on a silicon support. ( b ) Topography of a mixture of TMV and insulin aggregates on silicon. Scale bar, 500 nm. ( c ) Infrared near-field phase images ϕ 3 at two different frequencies, 1,634 cm −1 (left) and 1,660 cm −1 (right; 19 min total image acquisition time). ( d ) Nano-FTIR spectra of TMV (red, average of 70 interferograms; 19 min total acquisition time; 16 cm −1 resolution; × 4 zero filling) and insulin aggregate (green, average of 40 interferograms; 22 min total acquisition time; 8 cm −1 resolution × 4 zero filling). Red and green dots in the topography image mark the positions where the nano-FTIR spectra were taken. The position marked by the yellow dot and R indicates where the reference spectrum was recorded. ( e ) Map of TMV (purple) and insulin (yellow) aggregates. Full size image In Fig. 5a , we show attenuated total reflectance (ATR-)FTIR spectra of pure insulin aggregates (black curve) and of the insulin/TMV mixture (blue curve). Both pure insulin and insulin/TMV samples were deposited on a silicon support. The ATR-FTIR spectrum of the insulin/TMV mixture closely matches the ATR-FTIR spectrum of pure insulin and does not reveal the presence of TMV. The topographical image ( Fig. 5b ) of the mixture shows rod-like structures and aggregates of up to 32 nm in height. Still, TMV and insulin cannot be clearly discriminated. Figure 5c shows the near-field infrared phase images at 1,634 and 1,660 cm −1 , corresponding to the centre frequencies of the amide I band for β-sheet and α-helical structure, respectively [11] . In both infrared images, all structures show a distinct absorption contrast. As expected, the phase contrast to the substrate (that is, absorption) increases with particle height (that is, volume). Comparing the two infrared images, we find a significant increase of the phase contrast from 1,634 to 1,660 cm −1 for the smooth rod in the lower left corner of the image, while for all other structures the phase contrast did not change with respect to the substrate. From this observation, we conclude that α-helices form this rod-like structure, which is thus most probably a TMV. For identification of the secondary structure, we recorded nano-FTIR spectra ( Fig. 5d ) on the smooth rod at the position marked by the red dot in the topography image (red spectrum), and on the aggregate marked by the green dot (green spectrum). The red spectrum exhibits the absorption maximum at 1,660 cm −1 , which corresponds to the amide I resonance frequency of α-helices. Further, the shape fits well to the infrared spectrum of TMV ( Fig. 2d ). These results lead us to identify this rod-like structure as a TMV particle. In contrast, the green spectrum significantly differs from the red, exhibiting two peaks at 1,660 and 1,634 cm −1 , which are attributed to the presence of α-helices and β-sheets, respectively. Thus, we can identify this particle as an insulin aggregate, as its nano-FTIR spectrum agrees with the ATR-FTIR spectrum of the pure insulin sample ( Fig. 5a , black curve). Note that we compare the nano-FTIR spectrum with an ATR-FTIR spectrum, in contrast to Fig. 2 , as the infrared signal was too weak to obtain a GI-FTIR spectrum. As ATR-FTIR spectra are typically red shifted relative to GI-FTIR spectra [36] (see Supplementary Fig. S1 ), the ATR-FTIR spectrum is slightly red shifted compared with the nano-FTIR spectrum. To visualize the nanoscale distribution of TMV and insulin aggregates, that is, the nanoscale structural heterogeneity of the sample, we calculated the ratio between the infrared phase images at 1,660 and 1,634 cm −1 . From the spectra displayed in Fig. 5d , we know that the absorption of TMV is stronger at 1,660 than at 1,634 cm −1 . For insulin, the absorption is stronger at 1,634 cm −1 . Every image pixel where we obtain a ratio that is significantly larger than 1 thus reveals TMV. Pixel where we obtain a ratio that is smaller than 1 reveals insulin. Figure 5e shows a map where pixel with ratio larger than 1.5 are depicted in purple, and pixel with ratio smaller than 1 in yellow. The map clearly reveals the TMV (purple) and shows that all other protein structures (yellow) have a strong signal at 1,634 cm −1 , which can be attributed to the presence of β-sheets. This allows us to identify them as insulin aggregates. Nano-FTIR studies of individual insulin fibrils Having demonstrated the capability of mapping secondary structure on the nanometre scale, nano-FTIR is well prepared for applications in biochemical and biomedical research. We explore as a first application example the protein conformation in individual insulin fibrils ( Fig. 6 ). Insulin can form amyloid-like fibrils and fibres composed of filament-shaped protein aggregates [11] , [32] , [40] , which renders it an excellent and widely used model system for neurodegenerative disease research (that is, Alzheimer and Parkinson). Studies [32] , [41] show that the filaments have a core composed of β-sheets ( Fig. 6c ). It is assumed that this core is surrounded by randomly oriented secondary structures, including α-helices, β-turns and unordered structures [11] . However, the exact structure of the shell is still an open question of high biological relevance [40] . Recent studies by tip-enhanced Raman spectroscopy indicate the presence of α-helices/unordered structures at the surface of the fibrils [42] , [43] . In the following, we apply nano-FTIR to study the protein conformation in insulin fibrils. 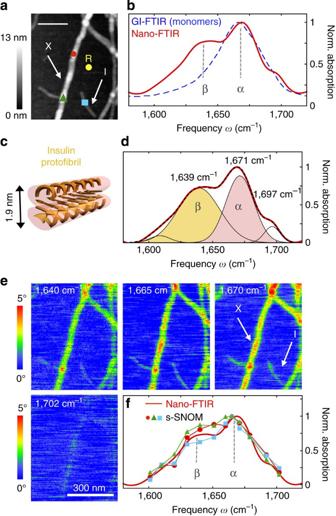Figure 6: Infrared nanospectroscopy and nanoimaging of secondary structure in individual insulin fibrils. (a) Topography of insulin fibrils on a silicon substrate. Scale bar, 200 nm. The arrows indicate a type I fibril (I) and a 9-nm-thick fibril composed of several protofilaments (X), respectively. (b) Nano-FTIR spectrum of a 9-nm-thick insulin fibril (red, average of 154 interferograms; 8 cm−1resolution; × 4 zero filling) recorded at the position marked by the red symbol ina. The position marked by the yellow dot and R indicates where the reference spectrum was recorded. The dashed blue line shows for comparison a GI-FTIR spectrum of insulin monomers on a gold substrate. (c) Illustration of the structure of an amyloid-like insulin protofibril (a type I fibril consists of two protofibrils). (d) Band decomposition of the nano-FTIR spectrum (red curve) based on five absorption bands (thin black curves). The dashed black curve shows the resulting fit. (e) s-SNOM phase images of the fibrils shown ina. Scale bar, 300 nm. (f) Local infrared absorption spectra (symbols) depicting the normalized imaginary part of the near-field signal at the positions marked ina. The data points were extracted from 12 near-field amplitude and phase images and were normalized to the imaginary part of the near-field signal on the silicon substrate. Four of the phase images are shown ine. For comparison, the nano-FTIR spectrum ofbis depicted by the red thick curve. All spectra are normalized to their maximum value. Figure 6: Infrared nanospectroscopy and nanoimaging of secondary structure in individual insulin fibrils. ( a ) Topography of insulin fibrils on a silicon substrate. Scale bar, 200 nm. The arrows indicate a type I fibril (I) and a 9-nm-thick fibril composed of several protofilaments (X), respectively. ( b ) Nano-FTIR spectrum of a 9-nm-thick insulin fibril (red, average of 154 interferograms; 8 cm −1 resolution; × 4 zero filling) recorded at the position marked by the red symbol in a . The position marked by the yellow dot and R indicates where the reference spectrum was recorded. The dashed blue line shows for comparison a GI-FTIR spectrum of insulin monomers on a gold substrate. ( c ) Illustration of the structure of an amyloid-like insulin protofibril (a type I fibril consists of two protofibrils). ( d ) Band decomposition of the nano-FTIR spectrum (red curve) based on five absorption bands (thin black curves). The dashed black curve shows the resulting fit. ( e ) s-SNOM phase images of the fibrils shown in a . Scale bar, 300 nm. ( f ) Local infrared absorption spectra (symbols) depicting the normalized imaginary part of the near-field signal at the positions marked in a . The data points were extracted from 12 near-field amplitude and phase images and were normalized to the imaginary part of the near-field signal on the silicon substrate. Four of the phase images are shown in e . For comparison, the nano-FTIR spectrum of b is depicted by the red thick curve. All spectra are normalized to their maximum value. Full size image In contrast to Fig. 5 , insulin fibrils were grown by incubating insulin protein at 60 °C in a pH 2 buffer for 30 h, thus representing a biologically relevant model system. In Fig. 6a , the topography of a sample area is shown where we found type I (3 nm high, consisting of two protofibrils, respectively four protofilaments, marked I) and thicker insulin fibrils (with increasing thickness the number of protofilaments increases) with heights ranging from 5 to 10 nm [11] , [44] , [45] . In the nano-FTIR spectrum of a 9-nm-thick fibril ( Fig. 6b , red curve, taken at the position marked by the red dot in the topographical image), we find the strongest peak at 1,669 cm −1 . By comparison with a GI-FTIR spectrum of monomeric insulin (predominantly α-helical structure, blue dashed curve), we can assign this peak to the presence of α-helices. The peak at 1,638 cm −1 is assigned to β-sheets. However, it is relatively weak compared with the nano-FTIR spectrum of the insulin aggregates ( Fig. 5 ). We explain this observation by the well-aligned β-sheet structure forming the core of the fibrils seen in Fig. 6 , where the dipole orientation of the amide I band is mostly parallel to the filament axes (that is, to the substrate surface) [13] , [46] . As seen before in Fig. 3 with PM, protein vibrations parallel to the substrate couple only weakly to the near field at the tip apex and thus are suppressed in the nano-FTIR spectra. Standard band decomposition of the nano-FTIR spectrum ( Fig. 6d ) reveals two major bands at 1,639 and at 1,671 cm −1 , confirming that β-sheet and α-helical structures are the predominant contributions. The band at 1,697 cm −1 could be caused by β-turns or even antiparallel β-sheet structure and the weak band at 1,609 cm −1 might indicate side chains. Most importantly, no band is observed in between the β- and α-peaks where typically disordered structure is located [10] . Thus, we conclude that disordered structures are almost absent in the fibrils. Note that the dipole of the amide I band is isotropically oriented in disordered structures and thus cannot be the cause for this observation. To explore the presence of α-helices in type I insulin fibrils (which are only 3 nm thick), we performed infrared s-SNOM imaging at different frequencies provided by our QCL. For nano-FTIR of such thin fibrils, the broadband laser source does not yet provide enough infrared power. Figure 6e shows infrared near-field phase images at four different wavelengths, exhibiting clear contrast for both type I and 9 nm thick fibrils. From altogether 12 images, we extracted local infrared spectra at the positions marked by the red, green and blue symbols in Fig. 6a . The spectra are plotted in Fig. 6f using the corresponding symbols. For both the 9-nm-thick fibril (red and green symbols) and type I (blue symbols) fibril, we find the same spectral signature as observed in the nano-FTIR spectrum (thick red curve in Fig. 6f ). The spectrum acquired at the position marked by the blue symbol in Fig. 6a thus provides experimental evidence that α-helices are also present in type I fibrils. The current resolution of about 30 nm does not allow for concluding whether the α-helices are inside the core or forming a shell. Assuming that the core is formed of purely β-sheets (according to current models [41] ), our findings suggest that the shell is highly structured (mainly α-helical structure) and not randomly organized. The presence of α-helices in the shell could explain the tendency of fibrils to associate. Nano-FTIR enables reliable probing and mapping of protein secondary structure with nanoscale resolution, and close to single-protein sensitivity. Our results indicate that infrared spectra of one ferritin complex can be obtained, which demonstrates extraordinary sensitivity of nano-FTIR to ultra-small amounts of material, in case of one ferritin complex 0.8 × 10 −18 g (about 1 attogram) of protein, respectively, 5,000 C=O bonds. By further sharpening the tips and optimizing their antenna performance [47] , we envision single-protein spectroscopy in the future, paving the way to a new era in infrared biospectroscopy. We foresee manifold applications, such as studies of conformational changes in amyloid structures on the molecular level, the mapping of nanoscale protein modifications in biomedical tissue or the label-free mapping of membrane proteins. To operate under physiological conditions, for example, to study the membrane of living cells, s-SNOM and nano-FTIR have to operate in liquids. Indeed, scanning near-field optical optical microscopy in liquids and under physiological conditions has been already demonstrated [48] , [49] . To perform nano-FTIR, the water could be exchanged by D 2 O, which is typically done in conventional FTIR to eliminate infrared absorption by H 2 O in the region of the amide I band [50] . s-SNOM The AFM is operated in dynamic mode, where a standard Au-coated tip (PPP-NCSTAu, Nanosensors) is vertically vibrating with an amplitude of about 40 nm at the mechanical resonance frequency Ω of the cantilever, in this work at about Ω~135 kHz. For infrared imaging, we use a QCL (Daylight Solutions, USA), tunable between 1,560 and 1,750 cm −1 . A Michelson interferometer is used to analyse the tip-scattered light. Unavoidable background signals can be efficiently suppressed by demodulating the detector signal at a higher harmonic of the tapping frequency, n Ω (ref. 34 ). Employing a pseudoheterodyne detection scheme [34] (where the reference mirror oscillates at a frequency M ) enables the simultaneous detection of both amplitude and phase signals. In all presented images, the demodulation order was n =3. The images were recorded with an integration time of 25 ms per pixel, resulting in a total image acquisition time of several minutes, depending on the number of pixel. nano-FTIR For broadband spectroscopy, the AFM tip is illuminated with a coherent mid-infrared beam of an average output power of about 100 μW (refs 16 , 17 , 35 ). The broadband mid-infrared laser beam is generated by a difference frequency generator (Lasnix, Germany) where two near-infrared, 100-fs pulse trains from a fibre-laser system (FemtoFiber pro IR and SCIR, Toptica Germany) are superimposed in a GaSe crystal. This mid-infrared source emits a continuous spectrum with a usable width up to 700 cm −1 , which can be tuned within the limits 700–2,500 cm −1 dependent on difference frequency generator settings (for example, the crystal orientation). FTIR spectroscopy of the light scattered by the tip is performed by recording the demodulated detector signal I as a function of the reference mirror position d . Because of the asymmetry of the interferometer (that is, the sample is located in one interferometer arm), Fourier transformation of the interferogram I ( d ) subsequently yields the near-field amplitude and phase spectra. In all presented nano-FTIR spectra, the demodulation order was n =3 except for the nano-FTIR spectra shown in Fig. 3 where it was n =2. As the sample stage is subject to unavoidable mechanical drift in the range of several nanometres per minute, we recorded individual interferograms of the object (TMV, ferritin, insulin aggregates and fibrils) with an acquisition time of 23 s. To improve the signal-to-noise ratio, the interferograms were recorded multiple times (the numbers of interferograms are provided in the figure captions) and an average was calculated. Between each of the nano-FTIR measurements, the tip was relocated to the original point on the object. Relocation was done with the help of topography images, which were recorded in between each interferogram acquisition. Subsequent Fourier transformation of the averaged interferograms yields the complex valued near-field spectra of the object, . For normalizing the spectra of the objects, the tip was positioned on a clean area of the silicon substrate close to the object and reference interferograms were recorded. We recorded a similar number of interferograms as on the object, each one in 23 s. Fourier transformation of the averaged interferograms yields the near-field reference spectrum , that is, the near-field spectrum of the clean silicon surface. By complex-valued division, E n ( ω )/ E ref ,n ( ω ), we obtained the normalized amplitude s n ( ω )/ s ref ,n ( ω ) and phase ϕ n ( ω )− ϕ ref ,n ( ω ) spectra of the object, yielding the nano-FTIR absorption spectra of the object, a n ( ω )= s n / s ref ,n sin ( ϕ n – ϕ ref ,n ). FTIR We used a Bruker Hyperion 2000 microscope coupled to a Vertex 70 FTIR spectrometer equipped with GI and ATR modules and a liquid-nitrogen-cooled mid-band mercury cadmium telluride detector. All FTIR spectra show the absorbance. The GI module ( × 15 GI reflection objective, Bruker) comprises a plane mirror that reflects the beam onto the sample surface at grazing angle incidence. The reflected beam is backreflected and refocused onto the same sample area and then collected and detected. The spectra were measured with a spectral resolution of 4 cm −1 and present an average over 1,000 scans with a total acquisition time of 860 s. All samples were prepared on a 150-nm-thick gold film on silicon. The reference spectra were recorded on a cleaned 150 nm thick gold film on a silicon wafer. The ATR module ( × 20 ATR objective, Bruker, single internal reflection) comprises a germanium crystal with a diameter of about 100 μm at the point of contact with the sample. The spectra were measured with a spectral resolution of 4 cm −1 and present an average over 1,000 scans with a total acquisition time of 860 s. The samples were prepared on a silicon wafer or on a gold-coated silicon wafer. The reference spectra were recorded on a cleaned silicon wafer or gold-coated silicon wafer, respectively. Decomposition of the amide I band The band decomposition was performed with the OPUS software package (version 4.2) supplied by Bruker. As a starting point for the curve-fitting procedure, five individual absorption bands were proposed at 1,638, 1,655, 1,667, 1,685 and 1,705 cm −1 , defining parallel β-sheets, unordered, α-helices, β-turn and antiparallel β-sheet structures, respectively. The curve fitting was successfully performed based on the damped least-squares optimization algorithm developed by Levenberg–Marquardt and assuming Gaussian band envelopes. The obtained residual root mean squared error was 0.0048. Comparing the nano-FTIR spectrum of the insulin fibrils with a GI-FTIR spectrum of insulin monomers (peak maximum at 1,666 cm −1 ), we can assign the peak at 1,671 cm −1 to α-helical structure. The insulin monomers are dominantly α-helical structure, as we confirmed by circular dichroism measurements shown in Supplementary Fig. S3 . The frequency difference between 1,666 and 1,671 cm −1 might be caused by the structural change from monomer to fibril structure or owing to the different sample support, which in nano-FTIR is silicon and in GI-FTIR is gold. We note that a peak frequency of 1,666 cm −1 for α-helical structure seems to be unusually high. However, it can be readily explained by the grazing-incidence FTIR modality. It is well known that GI-FTIR spectra can be significantly blue shifted compared with standard transmission FTIR spectra [36] . We demonstrate this phenomenon in the Supplementary Fig. S1 where we compare a standard transmission FTIR spectrum with the GI-FTIR spectrum of the insulin monomer sample. The peak in the transmission FTIR spectrum occurs at the much lower frequency 1,656 cm −1 , which matches literature data (ranging from 1,654 to 1,658 cm −1 (refs 50 , 51 , 52 )). Sample preparation All water was deionized ultrapure (18 MΩcm). Substrate surfaces were used as provided, but in some cases additionally cleaned by ultrasonication in acetone, isopropanol and water (each for 10 min), and blow dried with nitrogen. For all s-SNOM and nano-FTIR measurements, all samples were prepared on silicon wafers. For GI-FTIR measurements, gold substrates were used (150 nm of thermally evaporated gold deposited on a silicon wafer), while for ATR-FTIR measurements silicon or gold-coated silicon wafers were used. TMV samples TMV suspension: A suspension of TMV (strain vulgare ), purified from systemically infected tobacco plants ( Nicotiana tabacum cv Samsun nn ) was kindly provided by Professor C. Wege (University of Stuttgart, Germany). TMV was dialyzed against water in a 10-kDa Slide-A-Lyzer dialysis unit (Thermo Fisher Scientific), and diluted with water. TMV for s-SNOM: Ten microlitres of 1 μg ml −1 suspension was spin coated (spin coater SCI-20, Schaefer Technologie) on a cleaned silicon wafer and dried in air. TMV for GI-FTIR: Ten microlitres of 1 μg ml −1 suspension was spin coated on a gold wafer, and dried in air. Ferritin samples Ferritin solution: Horse spleen ferritin solution (44 mg ml −1 , Sigma-Aldrich) was diluted 500-fold with water. Ferritin for s-SNOM: A droplet of Ferritin solution was deposited on a silicon wafer and incubated for 2 min. Excess of solution was removed with filter paper (Sigma) and the sample was dried in air. Ferritin for GI-FTIR: Ferritin solution was first purified with a spin desalting column (7 K MWCO, Thermo Scientific) and followed with the procedure as above, but on a gold substrate. PM samples Halobacteria ( H. salinarum strain S9) were cultivated in high-salt pepton medium (10 g l −1 pepton, 4.3 M NaCl, 80 mM MgSO 4 , 27 mM KCl, 10 mM sodium citrate, pH 6.5) for 6 days. The collected cells were lysed by osmotic shock with distilled water. PM fragments were purified by fractionated centrifugation [53] . PM for s-SNOM: A 30-μl droplet of a buffer pH 7.8, containing 150 mM of KCl and 20 mM of Tris, was deposited on a silicon substrate and 0.2 μl of purified PM (6 mg ml −1 ) was added into the droplet. Fifteen microlitres of imaging buffer was subsequently added into the droplet to ensure maximum dispersion of previously added PMs. The resulting droplet was incubated on the silicon substrate for 25 min and then rinsed several times with water and dried in air. PM for GI-FTIR: Same sample preparation procedure as for s-SNOM, but a gold substrate was used and the PM was incubated for 40 min. Insulin aggregate samples Insulin aggregate solution: Dispersions were prepared solubilizing 20 mg dehydrated human insulin (Sigma-Aldrich) in 1 ml 1 mM HCl solution. The solution was then re-diluted in 10 mM HCl/KCl at 2 mg ml −1 , and incubated at 60 °C for 24 h in a thermomixer (Eppendorf), followed by 2 years storage at 4 °C. Insulin aggregates (+TMV) for s-SNOM: Ten microlitres of insulin aggregate solution was spin coated (as for TMV) on a silicon substrate, and rinsed with water. Ten microlitres of 1 μg ml −1 TMV suspension was then spin coated on the dried insulin aggregates. Insulin aggregates for ATR-FTIR: Twenty microlitres of insulin aggregate solution was deposited on a silicon wafer, dried and rinsed with water. Insulin fibril samples Insulin fibril solution: Dispersions were prepared as above, but incubated at 60 °C for 30 h. Insulin fibrils for s-SNOM: Ten microlitres of insulin fibril solution was spin coated on a silicon wafer and rinsed with water. Insulin monomer samples Insulin monomer solution: Dispersions were prepared as above, but without any incubation. Insulin monomer for GI-FTIR: Twenty microlitres of insulin monomer solution was spin coated on a gold substrate and rinsed with water. How to cite this article: Amenabar, I. et al. Structural analysis and mapping of individual protein complexes by infrared nanospectroscopy. Nat. Commun. 4:2890 doi: 10.1038/ncomms3890 (2013).